Robust antiferromagnetic coupling in hard-soft bi-magnetic core/shell nanoparticles The growing miniaturization demand of magnetic devices is fuelling the recent interest in bi-magnetic nanoparticles as ultimate small components. One of the main goals has been to reproduce practical magnetic properties observed so far in layered systems. In this context, although useful effects such as exchange bias or spring magnets have been demonstrated in core/shell nanoparticles, other interesting key properties for devices remain elusive. Here we show a robust antiferromagnetic (AFM) coupling in core/shell nanoparticles which, in turn, leads to the foremost elucidation of positive exchange bias in bi-magnetic hard-soft systems and the remarkable regulation of the resonance field and amplitude. The AFM coupling in iron oxide—manganese oxide based, soft/hard and hard/soft, core/shell nanoparticles is demonstrated by magnetometry, ferromagnetic resonance and X-ray magnetic circular dichroism. Monte Carlo simulations prove the consistency of the AFM coupling. This unique coupling could give rise to more advanced applications of bi-magnetic core/shell nanoparticles. The continuously increasing interest in bi-magnetic core/shell nanoparticles is already delivering numerous appealing effects, such as large exchange bias, tailored coercivities (spring magnets), tunable blocking temperatures, two-stage magnetization reversal, high resonance fields or proximity effects [1] , [2] , [3] , [4] , [5] , [6] , [7] , [8] . In fact, some of these novel properties have resulted in prospective applications of these materials in diverse fields as magnetic recording (enhanced blocking temperature) [6] , hard magnets (increased energy products) [2] , shielding (superior microwave absorption) [7] , magnetoresistive devices (enhanced magnetoresistance after field cooling) [8] , improved magnetocaloric materials [9] , magnetic resonance amplifiers [10] or in biomedical applications (optimized hyperthermia and magnetic resonance imaging) [11] , [12] . Importantly, in all these experimental core/shell nanoparticles studies only ferromagnetic (FM) coupling between the counterparts (i.e., the spins of the core and the shell are aligned parallel to each other) has been reported. Nevertheless, Monte Carlo simulations have already probed the effects of different types interface couplings, such as antiferromagnetic (AFM) (i.e., layers antiparallel to each other), from the theoretical point of view. These studies predict a range of novel effects such as positive exchange bias, compensation points or proximity effects [13] , [14] , [15] , [16] . Interestingly, diverse types of couplings have been reported for thin film bilayers and multilayers [17] , [18] , [19] , [20] , [21] , [22] and in particular the AFM one, cause numerous significant effects, which have given rise to crucial magnetic devices such as novel types of recording media, advanced read heads in hard disks, magnetic random access memories and biomedical sensors [23] , [24] , [25] . However, the lack of more advanced interface couplings in core/shell nanoparticles may be precluding the development of new ground-breaking applications that could exploit their envisioned potential as miniaturized devices. Here we demonstrate, for the first time, using diverse techniques, the existence of an interfacial AFM coupling in high quality (with coherent interface growth) ferrimagnetic (FiM) soft/hard and hard/soft core/shell nanoparticles based on iron and manganese oxides. Such AFM coupling leads to the presence of positive exchange bias, which has never been observed neither in core/shell nanoparticles nor in hard-soft thin film systems. Importantly, this novel robust coupling, which is independent of the core size or the core/shell morphology, results in an easy control of the sign of the exchange bias by means of the cooling field and of the resonance field. Morphological and compositional characterization For this study, two types of samples were synthesized using seeded-growth [26] : (i) an inhomogeneous Mn-oxide layer was deposited on Fe-oxide seeds (with two different diameters—samples CS1 and CS2) and (ii) a homogeneous Fe-oxide layer was grown on Mn-oxide seeds (sample CS3) (see Methods). The procedure leads to core/shell nanoparticles with average sizes of 13(1) (CS1), 19(2) (CS2) and 9(2) (CS3) nm as evidenced by the transmission electron microscopy (TEM) images in Fig. 1a–c (see Supplementary Fig. S1 for the corresponding TEM images of the seeds and the particle size distributions). The structural characterization at the bulk (X-ray diffraction, Supplementary Fig. S2 ) and the single particle (fast Fourier transform-High Resolution TEM, Supplementary Fig. S2 ) level reveals the presence of both cubic (iron-based oxides) and tetragonal (manganese-based oxides) spinel structures. The core/shell morphology of the nanoparticles is clearly evidenced by combining scanning TEM (STEM) with electron energy loss spectroscopy (EELS) mapping ( Fig. 1d–f ) [27] , [28] . The crystal quality of the nanoparticles is very high, and the interfaces between the Fe-oxide and the Mn-oxide are coherent ( Fig. 1g–i ). Note that the mechanism of the seeded growth as well as the possible parameters affecting the thermodynamics of the process are briefly described in the Supplementary Discussion [29] . Given the magnetic properties of iron and manganese oxides, magnetically, the nanoparticles are composed by FiM soft low magnetic anisotropy- (iron-based oxides) and hard large magnetic anisotropy (manganese-based oxides) phases [30] . 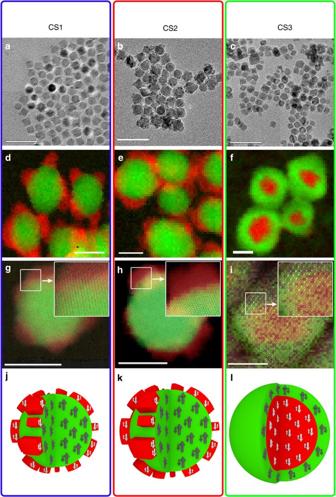Figure 1: Morphological and composition characterization. TEM images of the (a) CS1, (b) CS2 and (c) CS3 nanoparticles (scale bar=50 nm). EELS-mapping of the (d) CS1, (e) CS2 (scale bar=10 nm) and (f) CS3 (scale bar=5 nm) nanoparticles (where green corresponds to the Fe L signal and red to the Mn L edge, after background subtraction using a power law fit). High resolution-STEM annular dark field image overlaid with the EELS maps for the (g) CS1, (h) CS2 (scale bar=10 nm) and (i) CS3 (scale bar=5 nm) nanoparticles. Shown in the insets are enlarged views of the highlighted areas. Schematic representation of the morphological and magnetic structure for the (j,k) soft/hard and (l) hard/soft nanoparticles. Figure 1: Morphological and composition characterization. TEM images of the ( a ) CS1, ( b ) CS2 and ( c ) CS3 nanoparticles (scale bar=50 nm). EELS-mapping of the ( d ) CS1, ( e ) CS2 (scale bar=10 nm) and ( f ) CS3 (scale bar=5 nm) nanoparticles (where green corresponds to the Fe L signal and red to the Mn L edge, after background subtraction using a power law fit). High resolution-STEM annular dark field image overlaid with the EELS maps for the ( g ) CS1, ( h ) CS2 (scale bar=10 nm) and ( i ) CS3 (scale bar=5 nm) nanoparticles. Shown in the insets are enlarged views of the highlighted areas. Schematic representation of the morphological and magnetic structure for the ( j , k ) soft/hard and ( l ) hard/soft nanoparticles. Full size image Temperature dependence of the magnetization At high temperatures, the low field zero field cool (ZFC)-FC magnetization ( M ) curves ( Fig. 2a and Supplementary Fig. S3a,b ) exhibit the features of a blocking temperature ( T B ) (different for each sample) while at low temperature they show a second transition (independent of the type of particle). T B can thus be assigned to the Fe-oxide soft phase [30] , whereas the low temperature transition corresponds to the Curie temperature ( T C ) of the hard counterparts (Mn 3 O 4 , T C ~40 K). Remarkably, in contrast to conventional systems, below ~40 K, the magnetization exhibits a sharp decrease both for the FC and the ZFC curves. This feature persists up to moderately large fields (several Teslas; Fig. 2b and Supplementary Fig. S3a,b ). These results imply that when the manganese oxide orders magnetically at T C it must couple antiferromagnetically to the iron oxide [19] (see Fig. 1j–l ) resulting in the observed decrease in M . In fact, under some conditions M ( T ) is negative at low temperatures becoming positive as T is increased. Namely, at a given temperature magnetization of both phases cancels out, leading to a ‘compensation point’ (i.e., a zero net magnetization) [19] , similar to what has been predicted theoretically for core/shell nanoparticles [13] . Interestingly, upon increasing the field the magnetization progressively exhibits an upturn at T C (Mn-oxide) ( Fig. 2b ), indicating that the AFM coupling is gradually overcome for sufficiently large fields and eventually the spins become ferromagnetically aligned. Note that given the high quality of the interface ( Fig. 1g–l ), for simplicity, the core/shell coupling has been assumed as collinear, that is AFM at low fields ( Fig. 1j–l ) and FM at high fields. However, due to the effects related to the core/shell morphology (e.g., interface strains, surface anisotropy and shape anisotropy) and the known triangular spin structure in Mn 3 O 4 (ref. 31 ), the spins of the two phases, particularly at the interface, may exhibit more complex non-collinear structures as schematically shown in Supplementary Fig. S4 . However, the elucidation of the precise spin structures is beyond the scope of this article. 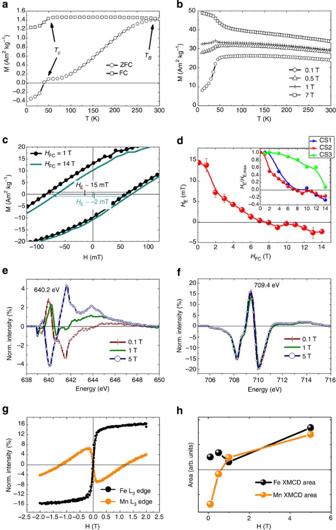Figure 2: Magnetic and dichroism characterization. (a) Low field FC-ZFC temperature dependence of the magnetization and (b), high field ZFC temperature dependence of the magnetization for the CS2 nanoparticles. (c) Enlarged hysteresis loops for the CS2 nanoparticles after FC in 1 T and 14 T. (d) Cooling field,HFC, dependence ofHEfor the CS2 nanoparticles. Shown in the inset is theHFCdependence of the normalizedHE,HE/HE,max, for the CS1, CS2 and CS3 nanoparticles. The error bars represent the error in the interpolation of the hysteresis loops. XMCD spectra at the (e) Mn-edge and (f) Fe-edge for the CS2 nanoparticles. (g) Element-specific hysteresis loop for the CS2 nanoparticle. (h) Area of the of the XMCD spectra as a function of the magnetic field for the Fe- and Mn-edges for the CS2 nanoparticles. Figure 2: Magnetic and dichroism characterization. ( a ) Low field FC-ZFC temperature dependence of the magnetization and ( b ), high field ZFC temperature dependence of the magnetization for the CS2 nanoparticles. ( c ) Enlarged hysteresis loops for the CS2 nanoparticles after FC in 1 T and 14 T. ( d ) Cooling field, H FC , dependence of H E for the CS2 nanoparticles. Shown in the inset is the H FC dependence of the normalized H E , H E / H E,max , for the CS1, CS2 and CS3 nanoparticles. The error bars represent the error in the interpolation of the hysteresis loops. XMCD spectra at the ( e ) Mn-edge and ( f ) Fe-edge for the CS2 nanoparticles. ( g ) Element-specific hysteresis loop for the CS2 nanoparticle. ( h ) Area of the of the XMCD spectra as a function of the magnetic field for the Fe- and Mn-edges for the CS2 nanoparticles. Full size image X-ray magnetic circular dichroism analysis Unambiguous proof for the AFM coupling stems from element-specific X-ray magnetic circular dichroism (XMCD) measurements. It can be clearly seen that while the spectra at the Fe-edge are virtually independent of the field, at the Mn-edge the spectra change sign at high fields ( Fig. 2f,e ). Remarkably, the spectra show that at low fields the Fe 3+ in octahedral positions in the Fe-oxide are AFM coupled to the Mn 2+ in tetrahedral sites in the Mn-oxide, which is the arrangement expected in normal ferrite spinels, probably indicating that the Mn-O-Fe superexchange at the interface is responsible for the AFM coupling. Notably, while an AFM coupling it is expected within the bulk structure of a ferrite spinel for certain transition metal ions, an interface AFM coupling between two spinel phases will largely depend not only on the composition but also on the crystal quality of the interface. In fact, interface interdiffusion or a weak coupling between core and shell may have precluded its observation in similar systems [5] , [30] , [32] , [33] . Thereby, the coherent growth between core and shell observed in samples CS1–CS3 is almost certainly crucial to observe the AFM coupling. This coupling becomes even more obvious when measuring the element-specific hysteresis loops at the maximum intensity peaks of the Fe- and Mn-edges spectra (709.4 eV and 640.2 eV, respectively) ( Fig. 2g ), where although both loops have the same H C (a clear indication of a strong exchange coupling [30] ), at low fields the magnetization of the manganese phase is inverted with respect to the iron phase one. At high fields, the magnetization at the Mn-edge gradually reorients, eventually becoming of the same sign as the one at the Fe-edge. Note that gradual increase of M at high fields for the Mn-edge loop is related to the triangular spin structure of Mn 3 O 4 (ref. 31 ). Additionally, the area under the XMCD spectra (proportional to the total magnetization) of the Fe-edge remains positive for all fields, whereas the Mn-edge one changes from negative to positive at approximately 1T. Field dependence of the magnetization The magnetometry hysteresis loop for the CS2 sample ( Fig. 2c and Supplementary Fig. S5a ) exhibits a smooth shape consistent with a strong exchange coupling [30] with a slow approach to saturation in concordance with the XMCD-loops. The saturation magnetization, M S , of CS2 is consistent with its core/shell structure taking into account the M S of the seeds and the M S of Mn 3 O 4 (see Supplementary Discussion on the M S calculations and Supplementary Fig. S6 ). Importantly, the hysteresis loops of all core/shell samples exhibit loop shifts, i.e., exchange bias, H E , in the field axis after FC in small fields ( H FC =1T) ( Fig. 2c and Supplementary Figs S3c,d and S5a ), where, as expected, H E depends on the sample morphology [1] , [34] , [35] . This is a well-known effect for exchange coupled AFM/FM systems, although it can also be found in coupled FM or FiM soft/hard systems [34] , [35] , [36] , [37] . Interestingly, for large cooling fields the loops shift to the opposite direction, i.e., H E changes sign, ( Fig. 2c,d and Supplementary Fig. S3c–f ). This effect, i.e., positive exchange bias, can be ascribed to an AFM coupling between layers [18] , [34] , hence further strengthening our magnetization and XMCD results. These results present the first report of positive H E on any hard-soft system, including thin films. Notably, for CS3 14T is not sufficient to invert H E , in concordance with the need of higher fields to obtain an increase of magnetization below T C (Mn-oxide) ( Supplementary Fig. S3f ), indicating that while the morphology does not play an important role in the existence of the AFM coupling, it probably determines its strength. In contrast to H E , the cooling field only affects weakly the coercivity ( H C — Supplementary Figs S3e,f and S5b ), indicating that H C is mainly governed by the intrinsic properties of the counterparts [12] rather than the AFM character of the coupling. Ferromagnetic resonance measurements Moreover, preliminary ferromagnetic resonance (FMR) measurements [38] at 9.5 GHz for samples CS1 and CS3 show that due to the AFM interface coupling, the ordering of the Mn 3 O 4 dramatically decreases the amplitude, A , of the FMR signal and significantly modifies the resonance field, H R , of the system ( Fig. 3 ). 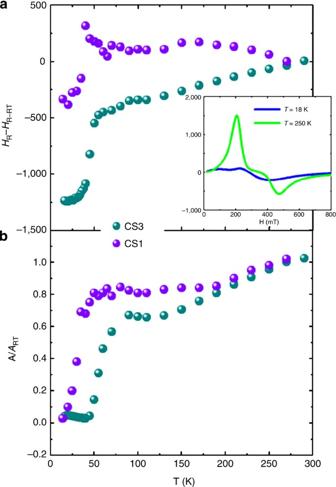Figure 3: Ferromagnetic resonance analysis. Temperature dependence of the (a) relative resonance position,HR, with respect to the room temperature resonance field (HR−RT) and (b) normalized amplitude,A, of the main resonance peak with respect to the room temperature amplitude,ART, for samples CS1 and CS3 at 9.5 GHz. Spectra at two temperature extremes for CS3 are shown in the inset. Figure 3: Ferromagnetic resonance analysis. Temperature dependence of the ( a ) relative resonance position, H R , with respect to the room temperature resonance field ( H R−RT ) and ( b ) normalized amplitude, A , of the main resonance peak with respect to the room temperature amplitude, A RT , for samples CS1 and CS3 at 9.5 GHz. Spectra at two temperature extremes for CS3 are shown in the inset. Full size image As can be seen in Supplementary Fig. S7a,b , at higher measuring frequencies (36.6 GHz) the samples show an analogous behaviour (i.e., with a sharp decrease in the resonance field and the amplitude) to that observed at 9.4 GHz, ruling out and frequency-related issues. Importantly, FMR measurements on the seed1 samples (i.e., the cores of CS1) show that pure Fe 3 O 4 nanoparticles exhibit smooth changes of H R and A with temperature ( Supplementary Fig. S7c ), implying that any features observed at low temperatures for the core/shell samples must be related to the presence of Mn 3 O 4 . Notably, the dramatic decrease in amplitude of the spectra at T C (Mn 3 O 4 ) occurs without any substantial increase in linewidth (inset of Fig. 3 ). This is a clear indication of a reduction of the overall magnetization at T C , in concordance with the magnetization measurements and consequently clear sign of AFM coupling. On the other hand, the significant drop in H R at the hard core ordering temperature clearly reflects that hard material ordering is noticeably changing the internal fields in the system. The interaction between the hard and soft systems can be understood as arising from an increased effective field at the Fe 3 O 4 counterpart due to the dipolar and exchange fields associated with the magnetization of the Mn 3 O 4 core and the AFM core/shell coupling. In fact, the hard-soft coupling could be used as a novel method to tune the resonance frequency of diverse magnetic systems. Finally, the fact the samples CS1 and CS3 exhibit similar behaviour strengthens our argument that while the AFM coupling is rather robust and does not depend on the morphology, the details of the coupling (e.g., its strength) may vary from sample to sample depending on their specific structure. Monte Carlo simulations Finally, Monte Carlo simulations for the soft/hard AFM coupled core/shell nanoparticles reproduce precisely the main experimental trends ( Fig. 4a ), i.e., the strong core/shell coupling and the different behaviour of the core and shell at high fields ( Fig. 4b ), the control over the sign of H E by the cooling field ( Fig. 4c ) as well as the direction of the magnetization of the shell ( Fig. 4d ). The simulations for the homogeneous hard/soft nanoparticles also have the same tendencies observed in experiments. Particularly, the sign reversal of H E occurs at considerably higher cooling fields ( Fig. 4c , inset), as observed experimentally. 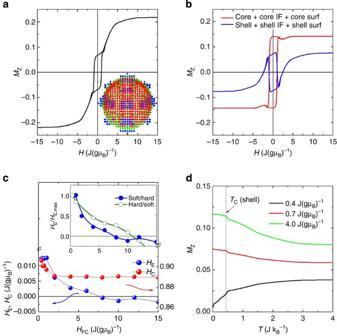Figure 4: Monte Carlo simulations. (a) Full hysteresis loop for the soft/hard nanoparticle. Shown in the inset is the structure used in the simulations. (b) Hysteresis loop corresponding to the core and the shell for the soft/hard nanoparticle. (c)HFCdependence ofHEandHCfor the soft/hard nanoparticle. Shown in the inset is theHFCdependence of the normalizedHEfor the soft/hard and the hard/soft nanoparticles. (d) Temperature dependence of the magnetization for the soft/hard nanoparticle for different applied fields. Figure 4: Monte Carlo simulations. ( a ) Full hysteresis loop for the soft/hard nanoparticle. Shown in the inset is the structure used in the simulations. ( b ) Hysteresis loop corresponding to the core and the shell for the soft/hard nanoparticle. ( c ) H FC dependence of H E and H C for the soft/hard nanoparticle. Shown in the inset is the H FC dependence of the normalized H E for the soft/hard and the hard/soft nanoparticles. ( d ) Temperature dependence of the magnetization for the soft/hard nanoparticle for different applied fields. Full size image In summary, we have unambiguously demonstrated the existence of a robust AFM coupling between core and shell in FiM soft/hard and hard/soft core/shell nanoparticles based on Fe-oxides and Mn-oxides. Furthermore, this AFM coupling has revealed for the first time the occurrence of positive exchange bias in any type of hard-soft system. Notably, the results reveal a simple and reversible, post-synthesis, way to tune the magnetic properties of the nanoparticles, i.e., without the need to alter their structural or morphological properties (e.g., size, composition or shape) as well as to control the resonance field and amplitude. In fact, the existence of an AFM interfacial coupling paves the way to more advanced applications of bi-magnetic core/shell nanoparticles as miniaturized versions of thin film devices for instance in spin dependent transport, spin filters, multilevel recording or magnetic encoders. Synthesis of the core/shell nanoparticles All starting materials were purchased from Sigma-Aldrich and used without further purification. The core/shell nanoparticles were synthesized following slightly modified seeded growth procedure reported earlier [26] , [30] . Synthesis of CS1 and CS2 nanoparticles: in a first step, spherical iron oxide nanoparticles were obtained by dissolving a given amount of iron (III) oleate and 1 mmol of oleic acid in 36 ml of 1-octadecene. The mixture was heated under magnetic stirring up to 320 °C (at 3 °C per min) and kept for 30 min. The slurry was removed from the heating source and allowed to cool down to room temperature. Two different surfactant-to-metal molar ratios, [S]/[M], of 0.6 and 1 were used, leading to iron oxide seeds of 10(1) (seed1) and 17(1) nm (seed2), respectively. In a second step, the iron oxide seeds were used to heterogeneously grow a manganese oxide layer. Briefly, a solution of 200 mg of iron oxide seeds and 50 ml of dibenzyl ether was degassed with several cycles of vacuum/argon gas at 100 °C. Subsequently, it was heated up to 220 °C, in which a solution containing 0.8 mmol (0.2 g) of manganese (II) acetylacetonate, 0.8 mmol of 1,2-hexadecanediol, 1.6 mmol of oleylamine, 0.6 mmol of oleic acid and 10 ml of dibenzyl ether was added at a fast injection rate. The slurry was maintained at 220 °C during 1 h under magnetic stirring after the fast injection. Finally, the reaction flask was removed from the heating source and cooled down in argon to room temperature. The procedure was repeated for the two iron oxide seeds (seed1 and seed2), resulting in two core/shell nanoparticles (CS1 and CS2). Both the iron oxide seeds and the core/shell nanoparticles were washed by several cycles of coagulation with ethanol, centrifugation at 2,000 g , disposal of supernatant solution and re-dispersion in hexane. Synthesis of CS3 nanoparticles: manganese oxide nanoparticle seeds (seed3) were synthesized by dissolving 1 g of manganese (II) acetylacetonate in 30 ml of oleylamine. The solution was degassed with several cycles of vacuum/argon gas at 100 °C and, then, slowly heated up to 210 °C and maintained at this temperature during 5 h. In a second step, the CS3 nanoparticles were obtained by dispersing 400 mg of manganese oxide seeds in 30 ml of dibenzyl ether, 0.6 mmol of iron (III) acetylacetonate, 2 mmol of 1,2-hexanedecandiol, 1.6 mmol of oleic acid and 1.7 mmol of oleylamine. The reaction flask was degassed with several cycles of vacuum/argon gas at 100 °C and heated to 250 °C during 20 min. Both the manganese oxide seeds and the core/shell nanoparticles were washed by several cycles of coagulation with ethanol, centrifugation at 2,000 g , disposal of the supernatant solution and re-dispersion in hexane. Structural and morphological characterization TEM images were obtained using a JEM-2100 with a LaB 6 filament. High resolution-scanning TEM and electron energy loss spectroscopy mapping have been obtained using an aberration-corrected Nion UltraSTEM100 operating at 100 kV and equipped with a Gatan Enfina EEL spectrometer and a X-FEG FEI TITAN operated at 300 kV fitted with a CEOS Probe Corrector and a Gatan Tridiem Energy Filter. X-ray diffraction patterns were collected using a Panalytical X’Pert Pro diffractometer with Cu Kα radiation. The measurements were carried out in a range of 10–65° in steps of 0.012° and collection time of 500 s. Magnetic measurements The magnetic properties of the nanoparticles were measured on tightly packed powdered samples using a superconducting quantum interference device magnetometer with 7 T maximum field and vibrating sample magnetometer with a maximum field of 14 T. The magnetization versus temperature measurements were performed in ZFC and FC conditions at different applied fields 1 mT, 5 mT, 1 T and 7 T. The hysteresis loops were carried out using a maximum field of 14 T after FC in diverse fields (in the range 0.2–14 T) from 300 K to 10 K. X-ray magnetic circular dichroism XMCD measurements were performed on dried core/shell nanoparticles spread onto carbon tape at the 4-ID-C beamline of the Advance Photon Source of the Argonne National Laboratory and the ID08 beamline of the European Synchrotron Radiation Facility (ESRF). XMCD spectra were recorded at the Fe and Mn L 2,3 edges using total electron yield mode at 10 K in different magnetic fields. The element resolved XMCD hysteresis loops, for the Fe and Mn L 3 edges, were acquired by recording the field dependence of the XMCD signal at the energies corresponding to three main peaks of the Fe-edge (i.e., 707.6, 708.7 and 709.4 eV) and for the main energy of the Mn-edge (640.2 eV). The XMCD signal was normalized by the area of the X-ray absorption spectra after correcting for the background. Note that since the Fe-edge loops at the different energies were analogous only the one at E =709.4 eV is used in the discussion. Ferromagnetic resonance measurements Fixed frequency—variable field ferromagnetic resonance (FMR) measurements were made at 9.4 GHz and 36.6 GHz in standard rectangular cavities. The temperature was varied using Oxford-Instruments flow-through cryostats. Monte carlo simulations We consider nanoparticles of a FiM1 soft core/FiM2 hard shell (with a total radius of R =14 lattice spacings) and of a FiM2 hard core/FiM1 soft shell (with a total radius of R =9 lattice spacings), on a simple cubic (sc) lattice. For the FiM1 soft core/FiM2 hard shell case, the spherical core has a radius R =10 lattice spacings. The shell thickness is t =4 lattice spacings. Following the TEM results, the shell has a special notched morphology made by asymmetrical patches on the core/shell interface leaving parts of core/shell interface bare creating the core surface (see inset in Fig. 3a ). For the FiM2 hard core/FiM1 soft shell case, the spherical core has a radius R =4 lattice spacings and a uniform shell of t =5 lattice spacings. The spins in the particle interact with nearest neighbours Heisenberg exchange interaction, and at each crystal site they experience a uniaxial anisotropy. In the presence of an external magnetic field, the total energy of the FiM1 soft core/FiM2 hard shell system is Here S i is the atomic spin at site i and ê i is the unit vector in the direction of the easy axis at site i. We consider the magnitude of the atomic spins in the two FiM sublattices to be equal to 1 and 1.4 in the core, the core interface (IF) and core surface (surf) and 1 and 0.5 in the shell, the shell IF and the shell surf. The first term gives the exchange interaction between the spins in the core, while the second term gives the exchange interaction in the shell. The critical temperature of Fe 3 O 4 is 20 times larger than the critical temperature of Mn 3 O 4 , thus we set the exchange coupling constant of the soft countepart J core =−30.0 J and of the hard material J shell =−1.5 J. The third term gives the exchange interaction at the interface between the core and the shell. The interface includes the last layer of the core and the first layer of the shell. The exchange coupling constant of the interface J IF is taken equal to J core . The forth term gives the anisotropy energy of the core, the core IF and the core surf. We consider K core = K core_IF= K core_surf =0.01 J. The fifth term gives the anisotropy energy of the shell IF, the shell and the shell surface, K shell_surf =1.2 J and K shell = K shell_IF =0.05 J. The core, the core IF, the shell and the shell IF anisotropies are uniaxial and directed along the z axis. The core_surf and the shell_surf anisotropies are taken as radial. The last term is the Zeeman energy. Analogous parameters were used for the FiM2 hard core/FiM1 soft shell case. The only difference is in the magnitude of the shell_surf anisotropy, which is taken equal to 0.05 J, due to the smaller size of the nanoparticles. We perform our simulations on isolated FiM core/shell nanoparticles using the Monte Carlo simulation technique with the implementation of the Metropolis algorithm [16] , [39] . The hysteresis loops are calculated after a field cooling procedure starting at temperature T =5.0 J k B −1 down to T =0.005 J k B −1 , at a constant rate under a static magnetic field H FC directed along the easy axis (i.e., the z axis). The hysteresis loop shift along the field axis, i.e., the exchange bias field, is given by H E =−( H right + H left )/2. The coercive field is defined as H C =( H right − H left )/2. H right and H left are the points where the loop intersects the field axis. The fields H , H C and H E are given in units of J(gμ B ) −1 , the temperature T in units J k B −1 and the anisotropy coupling constants K in units of J, where J is the exchange coupling constant of a ferromagnet and is taken equal to 1. The ZFC magnetization curves are calculated in the presence of a static field at a constant temperature rate. We have used 10 4 MC steps per spin (MCSS) at each field step d H =0.2 J (gμ B ) −1 and at each temperature step d T =0.25 J k B −1 , after discarding 2,500 MCSS for thermalization, to calculate the thermal average of magnetization. The results were averaged over 40 different samples (i.e., different random numbers). How to cite this article: Estrader, M. et al. Robust antiferromagnetic coupling in hard-soft bi-magnetic core/shell nanoparticles. Nat. Commun. 4:2960 doi: 10.1038/ncomms3960 (2013).